Photonic effects on the Förster resonance energy transfer efficiency Förster resonance energy transfer (ET) between luminescent species is applied in bio-imaging, lighting and photovoltaics, and has an important role in photosynthesis. However, the fundamental question of whether ET rates and efficiencies can be tuned by the photonic environment remains under debate. Here we show that ET rates are independent of the photonic environment, using the model system of LaPO 4 nanocrystals co-doped with Ce 3+ donors and Tb 3+ acceptors. Although the radiative emission rate of the Ce 3+ excited state increases with the refractive index of the solvent in which the nanocrystals are dispersed, the Ce 3+ -to-Tb 3+ ET rate does not. We demonstrate that, as a result, lower refractive index solvents enable higher ET efficiencies leading to higher Tb 3+ emission intensities. Furthermore, an analytical model for ET in (nano)crystalline host materials is presented, able to predict the dependence of ET efficiencies on the photonic environment and the concentration of acceptor ions. Tuning of spontaneous emission by photonic crystals, plasmonic nanostructures or dielectric cavities, has been a field of intense research [1] , [2] , [3] , [4] . Key is control over the local density of optical states (LDOS), which is directly proportional to the radiative emission rate. On the other hand, there have been few reports about photonic effects on Förster resonance energy transfer (ET) between luminescent centres. This type of ET is important in photosynthesis [5] , [6] , as well as for the operation of devices such as fluorescent tubes and solid state lasers. It also lies at the core of emerging technologies such as background-free bio-imaging [7] , [8] , and spectral conversion for increased solar cell efficiencies [9] . Tunability of ET would allow for precise control over energy flow and spectral output of luminescent materials. Unfortunately, previous studies disagree on the most fundamental question of how ET rates scale with the LDOS. De Dood et al. [10] and Blum et al. [11] find that ET rates are independent of the LDOS, whereas other works claim a linear [12] , [13] , or even a quadratic [14] dependence. The contradictory findings reported thus far may in part result from the complexity of the experimental systems used. The decay dynamics of the donor were measured in layered structures with (varying) distance between donor–acceptor pairs and an interface. Some studies compared separately fabricated samples [12] , [11] , which is not ideal because reproducible control over the thickness and refractive index of the spacer layers can be difficult. In other cases, energy migration among donors and transfer to multiple acceptors [10] , [12] , [13] , [14] would lead to non-exponential decay dynamics which are hard to interpret. In this work we quantify the ET in co-doped LaPO 4 nanocrystals (NCs), for different photonic environments and acceptor concentrations. Co-doped NCs are an ideal model system to study the influence of the LDOS on the ET rate. The crystallinity of the host material ensures that the donor–acceptor distances and the local electronic environment of the luminescent ions are well defined and fixed. At the same time, the photonic environment can be varied easily by dispersing the NCs in solvents with different refractive indices. A complicating factor is that random substitutional doping leads to an ensemble of donor ions with a different number of and separation from nearby acceptors. However, it is possible to accurately model the ET dynamics in a crystalline environment under the assumption of random donor and acceptor positions [15] , [16] . We measure the decay dynamics of the Ce 3+ excited state as a function of the concentration of Tb 3+ acceptor ions, and with the NCs dispersed in various solvents. Using a simple comparative method, we find that the radiative emission rate of the Ce 3+ excited state scales with the LDOS, whereas the Ce 3+ -to-Tb 3+ ET rate is independent. This finding is confirmed by more detailed analysis of the experimental decay dynamics using a model of ET in NCs. We furthermore show that, consequently, the efficiency of ET is higher if the LDOS is lower. This effect results in a higher Tb 3+ emission intensity if the NCs are dispersed in a solvent of lower refractive index. Our results demonstrate that the photonic environment can change the efficiency of ET, allowing for control over the energy flow and colour output of luminescent materials. Decay dynamics and emission spectra Our model system is schematically depicted in Fig. 1a : LaPO 4 NCs of 4 nm diameter doped with 1% Ce 3+ (purple; donor ions), and with varying Tb 3+ concentration (green; acceptor ions). 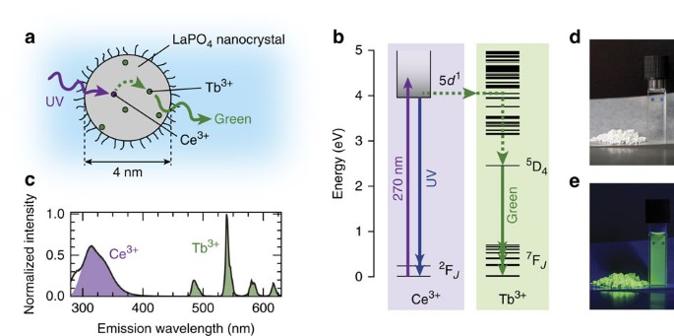Figure 1: Relaxation pathways in LaPO4nanocrystals co-doped with Ce3+and Tb3+. (a) LaPO4NCs with an average diameter of 4 nm are co-doped with Ce3+(purple) and Tb3+(green). A UV excited Ce3+centre can transfer its energy to a nearby Tb3+ion, resulting in emission in the visible. (b) Energy level diagram: absorption of a UV photon (purple arrow) brings Ce3+in the 5d1configuration. Subsequently, it can either radiatively decay to the 4f1ground configuration (blue arrows), or transfer its energy to a Tb3+acceptor (dashed green arrow). Tb3+rapidly relaxes to the5D4metastable state, followed by radiative decay to the7FJground state under the emission of a visible photon (solid green arrows). (c) The emission spectrum of LaPO4:Ce3+(1%)Tb3+(5%) NCs upon excitation in the Ce3+:4f1→5d1transition at 280 nm. The relative intensity of Ce3+:5d1→4f1(purple) and Tb3+:5D4→7FJ(green) emissions is determined by the ratio between the radiative emission rate and the energy transfer rate of the Ce3+:5d1excited state. Around 300 nm there is background emission from organic by-products of the NC synthesis. (d) A photograph in ambient light of LaPO4:Ce3+(1%)Tb3+(20%) NCs as a dried powder (left), and as a transparent NC dispersion in methanol (right). (e) The same NC powder (left) and dispersion (right) under UV excitation luminesce green. Figure 1b presents the energy level diagram of the Ce 3+ –Tb 3+ donor–acceptor pair [17] , [18] . After UV excitation of a Ce 3+ ion to the 5 d 1 state (purple arrow), it can either decay radiatively (blue arrows), or resonantly transfer its energy to a nearby Tb 3+ acceptor ion (green dashed arrow). Subsequently, Tb 3+ emits a visible photon in the transition from the 5 D 4 metastable state to one of the sublevels of the spin-orbit split 7 F J ground state. This gives rise to an emission spectrum as shown in Fig. 1c , containing a Ce 3+ emission band in the UV (300–360 nm) and several narrow emission lines in the visible (470–630 nm) from Tb 3+ . As shown in Fig. 1d,e for methanol, the NCs form a transparent dispersion in many polar solvents, which exhibits green luminescence under UV excitation. Figure 1: Relaxation pathways in LaPO 4 nanocrystals co-doped with Ce 3+ and Tb 3+ . ( a ) LaPO 4 NCs with an average diameter of 4 nm are co-doped with Ce 3+ (purple) and Tb 3+ (green). A UV excited Ce 3+ centre can transfer its energy to a nearby Tb 3+ ion, resulting in emission in the visible. ( b ) Energy level diagram: absorption of a UV photon (purple arrow) brings Ce 3+ in the 5 d 1 configuration. Subsequently, it can either radiatively decay to the 4 f 1 ground configuration (blue arrows), or transfer its energy to a Tb 3+ acceptor (dashed green arrow). Tb 3+ rapidly relaxes to the 5 D 4 metastable state, followed by radiative decay to the 7 F J ground state under the emission of a visible photon (solid green arrows). ( c ) The emission spectrum of LaPO 4 :Ce 3+ (1%)Tb 3+ (5%) NCs upon excitation in the Ce 3+ :4 f 1 →5 d 1 transition at 280 nm. The relative intensity of Ce 3+ :5 d 1 →4 f 1 (purple) and Tb 3+ : 5 D 4 → 7 F J (green) emissions is determined by the ratio between the radiative emission rate and the energy transfer rate of the Ce 3+ :5 d 1 excited state. Around 300 nm there is background emission from organic by-products of the NC synthesis. ( d ) A photograph in ambient light of LaPO 4 :Ce 3+ (1%)Tb 3+ (20%) NCs as a dried powder (left), and as a transparent NC dispersion in methanol (right). ( e ) The same NC powder (left) and dispersion (right) under UV excitation luminesce green. 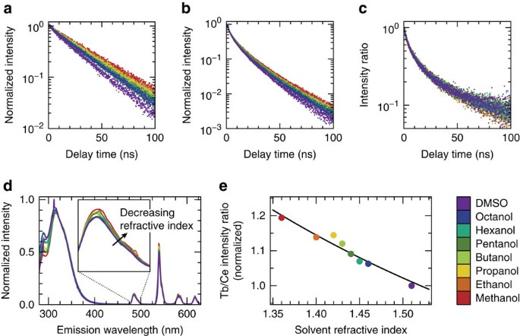Figure 2: The effects of an energy transfer rate independent of the photonic environment. (a) PL decay curves of the Ce3+emission (at 340 nm) from LaPO4:Ce3+(1%) NCs dispersed in solvents of different refractive index, ranging from 1.36 for methanol (red) to 1.51 for DMSO (purple). Note that decay is purely radiative as ET is impossible in the absence of Tb3+acceptor ions. (b) PL decay curves for LaPO4:Ce3+(1%)Tb3+(20%) NCs, in which efficient ET to Tb3+is possible. (c) Dividing the PL decay curve ofbby the radiative decay ofareveals the contribution of ET. We can see its independence of the refractive index of the solvent. (d) Emission spectra of LaPO4:Ce3+(1%)Tb3+(2%) NCs normalized to the Ce3+:5d1→4f1emission intensity (between 310 nm and 400 nm), in different solvents. The inset is a zoom of the5D4→7F6emission line. (e) A plot of the intensity ratio between Tb3+emission (470–630 nm) and Ce3+emission (310–400 nm) as a function of the solvent refractive index shows the 19% increase upon going from DMSO (n=1.51) to methanol (n=1.36). The solid black line depicts a good correspondence to the trend expected from equation 4. Full size image Figure 2a shows photoluminescence (PL) decay curves of the Ce 3+ emission for LaPO 4 :Ce 3+ (1%) NCs dispersed in different solvents. The decay dynamics are single-exponential and are faster in solvents with a higher refractive index, reflecting that the radiative emission rate scales with the LDOS. The PL decay curves for LaPO 4 :Ce 3+ (1%)Tb 3+ (20%) NCs are shown in Fig. 2b . They are non-exponential, as different Ce 3+ centres in the ensemble have different ET rates determined by the number and proximity of neighbouring Tb 3+ acceptors. Nevertheless, the trend of faster decay for higher refractive index is still visible. Figure 2: The effects of an energy transfer rate independent of the photonic environment. ( a ) PL decay curves of the Ce 3+ emission (at 340 nm) from LaPO 4 :Ce 3+ (1%) NCs dispersed in solvents of different refractive index, ranging from 1.36 for methanol (red) to 1.51 for DMSO (purple). Note that decay is purely radiative as ET is impossible in the absence of Tb 3+ acceptor ions. ( b ) PL decay curves for LaPO 4 :Ce 3+ (1%)Tb 3+ (20%) NCs, in which efficient ET to Tb 3+ is possible. ( c ) Dividing the PL decay curve of b by the radiative decay of a reveals the contribution of ET. We can see its independence of the refractive index of the solvent. ( d ) Emission spectra of LaPO 4 :Ce 3+ (1%)Tb 3+ (2%) NCs normalized to the Ce 3+ :5 d 1 →4 f 1 emission intensity (between 310 nm and 400 nm), in different solvents. The inset is a zoom of the 5 D 4 → 7 F 6 emission line. ( e ) A plot of the intensity ratio between Tb 3+ emission (470–630 nm) and Ce 3+ emission (310–400 nm) as a function of the solvent refractive index shows the 19% increase upon going from DMSO ( n =1.51) to methanol ( n =1.36). The solid black line depicts a good correspondence to the trend expected from equation 4. Full size image The PL decay curves in Fig. 2a,b can be used as direct proof that ET rates are independent of the LDOS. The donors in the ensemble have equal radiative emission rates γ rad but differ in ET rate. Hence, the decay dynamics of the ensemble can be factorized as where I ( t ) is the emission intensity at delay time t after an excitation pulse. The factor T ( t ) describes the decay due to ET, which is in general non-exponential. If we divide the non-exponential PL decay curve of Fig. 2b by the exponential decay dynamics as measured in the absence of Tb 3+ acceptors ( Fig. 2a ), we directly obtain the contribution of ET T ( t ). We plot T ( t ) in Fig. 2c for the different solvents. The trend of faster decay with increasing refractive index, which was visible in Fig. 2a,b , is no longer present. From this simple analysis we can already conclude that the trend observed in Fig. 2b is solely due to a dependence of the radiative emission rate on the LDOS, while the ET rate is independent. If indeed radiative decay and ET rates scale differently with the LDOS, then the ET efficiency should be tunable by the refractive index of the solvent [11] . More precisely, Ce 3+ -to-Tb 3+ ET becomes more efficient when competing radiative decay of the Ce 3+ excited state is suppressed. Hence, the Tb 3+ intensity should increase when we reduce the solvent refractive index. This is exactly what we observe. Figure 2d shows the emission spectra of LaPO 4 :Ce 3+ (1%)Tb 3+ (2%) NCs dispersed in different solvents. Upon going from dimethyl sulphoxide (DMSO; refractive index n =1.51) to methanol ( n =1.36), the relative Tb 3+ intensity increases by 19% ( Fig. 2e ). Modelling energy transfer in nanocrystals We now present an analytical model that reproduces how the decay dynamics of LaPO 4 :Ce 3+ (1%)Tb 3+ ( x %) NCs depend on x , and can be used to predict ET efficiencies in different photonic environments. For an isolated donor–acceptor pair at separation r having dipole–dipole interaction, the ET rate is γ ET = c / r 6 (ref. 19 ) with c the ‘ET strength’. The total decay rate Γ of a particular donor depends on the proximity of acceptors: where the summation runs over all (nearby) acceptors, and r i is the distance to acceptor i . In a crystal, only discrete donor–acceptor distances are possible, determined by the crystal lattice. For example, around the central donor ion in the schematic crystal of Fig. 3a , there is a ‘shell’ with n 1 =2 cation sites at distance r 1 (squares), one with n 2 =4 cation sites at distance r 2 (disks), and so on. Previously, our group has used this ‘shell model’ to simulate ET dynamics in a co-doped bulk crystal [15] , [16] . 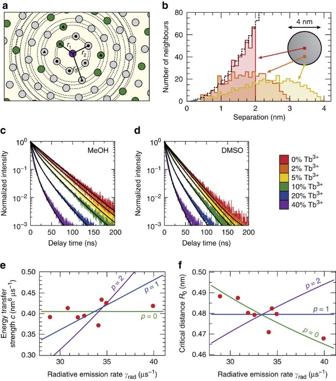Figure 3: The shell model for energy transfer in a (nano)crystalline environment. (a) Schematic of a doped crystal with cation sites (circles) on regular positions. Energy donor ions (purple) and acceptor ions (green) are randomly distributed. Around a donor ion there are discrete ‘shells’ (dashed circles) of cation sites at distances {r1,r2,r3,…}. These shells have space for a maximum of {n1,n2,n3,…} acceptor ions. The total ET rate of a central donor ion is set by the actual occupation of nearby shells. (b) The distribution of distances to nearby cation sites from a central (donor) ion, in a LaPO4NC with a diameter of 4 nm and with the central ion positioned at different depths from the NC surface (indicated by symbols in the inset). The distance distribution in a LaPO4NC is determined by the discrete nature of the crystal lattice, and by its finite size. For comparison, the black dashed line shows the distance distribution in a hypothetical glass-like continuous bulk material of the same density. (c,d) The decay dynamics of the Ce3+excited state in LaPO4:Ce3+(1%)Tb3+(x%) NCs withx={0, 2, 5, 10, 20, 40} (red, orange, yellow, green, blue, purple) dispersed in (c) methanol, and (d) DMSO. Solid lines are global fits to equation 3 (with account for the finite NC size), yielding a single value per solvent for the ET strengthc. (e) The ET strengthcand (f) the critical distanceR0against the radiative emission rate (which is proportional to the LDOS), obtained from fits as shown incandd. Solid lines are trends expected for three different scenarios; green: ET is independent of the LDOS, blue: ET scales linearly, and purple: ET scales quadratically. In the Methods section we show that under the assumption of a random distribution of donor and acceptor ions, the PL decay trace of an ensemble of donors in a bulk crystal can be written as: Figure 3: The shell model for energy transfer in a (nano)crystalline environment. ( a ) Schematic of a doped crystal with cation sites (circles) on regular positions. Energy donor ions (purple) and acceptor ions (green) are randomly distributed. Around a donor ion there are discrete ‘shells’ (dashed circles) of cation sites at distances { r 1 , r 2 , r 3 ,…}. These shells have space for a maximum of { n 1 , n 2 , n 3 ,…} acceptor ions. The total ET rate of a central donor ion is set by the actual occupation of nearby shells. ( b ) The distribution of distances to nearby cation sites from a central (donor) ion, in a LaPO 4 NC with a diameter of 4 nm and with the central ion positioned at different depths from the NC surface (indicated by symbols in the inset). The distance distribution in a LaPO 4 NC is determined by the discrete nature of the crystal lattice, and by its finite size. For comparison, the black dashed line shows the distance distribution in a hypothetical glass-like continuous bulk material of the same density. ( c , d ) The decay dynamics of the Ce 3+ excited state in LaPO 4 :Ce 3+ (1%)Tb 3+ ( x %) NCs with x ={0, 2, 5, 10, 20, 40} (red, orange, yellow, green, blue, purple) dispersed in ( c ) methanol, and ( d ) DMSO. Solid lines are global fits to equation 3 (with account for the finite NC size), yielding a single value per solvent for the ET strength c . ( e ) The ET strength c and ( f ) the critical distance R 0 against the radiative emission rate (which is proportional to the LDOS), obtained from fits as shown in c and d . Solid lines are trends expected for three different scenarios; green: ET is independent of the LDOS, blue: ET scales linearly, and purple: ET scales quadratically. Full size image Here, the product runs over all shells, and x ͛[0,1] is the acceptor concentration. The finite size of our NCs requires an adjustment to equation 3. As plotted in Fig. 3b , a donor ion close to the NC surface has fewer nearby cation sites than a donor ion in the centre. To account for these finite-size effects we consider the different possible donor positions in the NCs. For each position, we introduce a geometrical factor f i depending on the proximity of the NC surface: n i → f i n i (see Methods). Figure 3c,d shows the PL decay curves for LaPO 4 :Ce 3+ (1%)Tb 3+ ( x %) NCs with increasing x , in (c) methanol ( n =1.36) and (d) DMSO ( n =1.51). Supplementary Fig. 1 shows the decay dynamics in other solvents. Solid black lines are a global fit of the data for a specific solvent to our ET formula (equation 3), accounting for the finite size of a spherical NC with 4 nm diameter. Our model captures how the decay dynamics become faster and more non-exponential as the Tb 3+ concentration increases. Supplementary Fig. 2 demonstrates that neglecting finite-size effects leads to poor fits, especially at high acceptor concentrations. These fits to the decay dynamics allow us to extract the dependence of the ET strength c on the LDOS. They further confirm that γ rad scales with the solvent refractive index as expected (see Supplementary Fig. 3 ; in a separate publication we will discuss in more detail the effect of the solvent refractive index on the radiative decay of doped NCs [20] ). In Fig. 3e we plot the ET strength c against the LDOS (which scales linearly with γ rad ). Each data point corresponds to a different solvent, and depicts results of a global fit as in Fig. 3c,d . Solid lines give the trends expected for the three possibilities for the power p of the LDOS dependence of ET rates [12] , [13] , [14] . The fitted values of c are roughly constant with changing LDOS, at 0.405±0.021 nm 6 μs −1 . The linear or quadratic trends expected for p =1 (blue line) or p =2 (purple line) are absent. Hence, these fit results confirm our conclusion from Fig. 2 that ET rates are independent of the LDOS. As an alternative visualization, in Fig. 2f we plot the critical ET distance R 0 versus γ rad [11] . By definition R 0 =( c / γ rad ) 1/6 is the donor–acceptor separation at which there is 50% probability of ET. We see that R 0 becomes smaller with increasing LDOS, in agreement with the trend expected for p =0 (green line). With the fitted values of the (variable) radiative rate and the constant ET strength, we can use our analytical model to calculate the Ce 3+ -to-Tb 3+ ET efficiency η ET for NCs embedded in different photonic environments [21] : where again accounting for finite-size effects is needed in a nanocrystalline host. Figure 2e shows that equation 4 reproduces the observed increase of the Tb 3+ emission intensity in solvents of decreasing refractive index. Finally, using our model and our finding that the ET strength is a constant, we can predict ET efficiencies in more complex photonic environments than a homogeneous dielectric. For example, a photonic crystal structure inhibiting radiative decay by a factor 10 (ref. 4 ) can be used to increase the ET efficiency in LaPO 4 :Ce 3+ (1%)Tb 3+ (2%) NCs to 30% (now, 11–13% depending on the solvent). Conversely, co-doped NCs could be used as local probes for the LDOS in photonic structures, where the relative emission intensities of the dopants reveal the LDOS-dependent ET efficiency between them. Our results demonstrate that photonic structures developed for spontaneous emission control can have an important role in tuning the efficiency of ET. The concept of ET from sensitizers such as colloidal semiconductor quantum dots [22] , [23] , [24] , dye molecules [25] , [26] , [27] , [28] or silicon NCs [29] , [30] , [31] is widely used. It can, for example, improve the spectral response of photovoltaic devices, increase the output of phosphors or optical amplifiers or be used for colour tuning in lighting. Furthermore, ET has a crucial role in photon upconversion [28] , [32] , [33] used in bio-imaging and for next-generation photovoltaics. We envision that these and other applications can benefit from photonic enhancements of the ET efficiency. Synthesis and characterization We synthesized LaPO 4 NCs co-doped with Ce 3+ and Tb 3+ using the method of Oertel et al. [17] . Briefly, a clear solution of 10 mmol of lanthanide chlorides (La, Ce, Tb) in 10 ml of methanol was mixed with 40 mmol of diethyl ethylphosphonate. Methanol was evaporated under vacuum at room temperature, after which 30 ml of diphenyl ether was added. Following the removal of water under vacuum at 105 °C, we added 40 mmol of tributylamine and 7 ml of a 2 M solution of phosphoric acid in dihexyl ether. Subsequently, the reaction mixture was kept overnight under nitrogen at 200 °C, during which the NCs were formed. They were isolated by centrifugation, washed with toluene and dried under vacuum. From transmission electron microscopy ( Supplementary Fig. 4a ), we know that the NCs have a diameter of 4 nm and a polydispersity of 10%. Powder X-ray diffraction ( Supplementary Fig. 4b ) confirms that the NCs exhibit the monazite crystal structure of LaPO 4 up to the highest doping concentration of 40% Tb 3+ . The doping concentrations of 1% Ce 3+ , and a varying concentration (0, 2, 5, 10, 20, 40%) of Tb 3+ were confirmed using inductively coupled plasma atomic emission spectroscopy. Experimental details Photoluminescence measurements were performed using an Edinburgh Instruments FLS920 fluorescence spectrometer. For recording emission spectra we used a 450 W Xe lamp as excitation source and a Hamamatsu R928 PMT with a grating blazed at 300 nm for detection. For PL decay measurements, we used a PicoQuant PDL 800-B+PLS 8-2-409 pulsed diode laser emitting at 270 nm with a repetition rate of 2.5 MHz, and a Hamamatsu H74220-60 PMT with a grating blazed at 300 nm. To obtain the refractive index in the UV of the different solvents, we used a home-built setup to measure the critical angle of total internal reflection of a UV laser beam (Kimmon He/Cd IK3151R-E; λ =325 nm) on the glass/solvent interface. We found refractive indices of 1.36 for methanol, 1.40 for ethanol, 1.42 for 1-propanol, 1.43 for 1-butanol, 1.44 for 1-pentanol, 1.45 for 1-hexanol, 1.46 for 1-octanol and 1.51 for DMSO. Modelling the ET dynamics We consider an excited donor ion in a crystalline environment with acceptors randomly substituted, as expected in LaPO 4 :Ce 3+ , Tb 3+ from the chemical similarity of ions in the lanthanide series. Each nearby cation site has an independent probability x (the overall acceptor concentration) to contain an acceptor ion, hence add to the decay rate or, equivalently, a factor to the decay trace of the donor (with r j the separation from the donor). The decay trace of the ensemble of donors contains contributions from all possible donor environments: where the product runs over all (nearby) cation sites, and each factor accounts for a probability x that cation site j adds a decay component and a probability 1− x that it does not. Using the crystalline nature of the host we can write the above equation in terms of shells (see Fig. 3a ) [16] , leading to equation 3. As the ET rate rapidly decreases with increasing donor–acceptor separation (as r −6 ), we capture more than 99.5% of the ET when taking into account only the first 378 cation sites within 1.9 nm from the donor. We neglect the possibility of donor-to-donor energy migration, justified by the low donor concentration of 1%. This effect, however, may explain small deviations between the experimental decay dynamics and our model. Accounting for the finite size of a nanocrystal As depicted in Fig. 3b , donors close to the NC surface have a different crystalline environment than those near the centre. Assuming spherical NCs, we multiply the exponents n i in equation 3 by a geometrical factor where h is the radial coordinate of the donor ion and a is the NC radius. We take into account the possible donor positions in a spherical NC by summation of equation 3 over different values of h with h 3 evenly distributed over the interval [0, a 3 ]. We must, however, note that the actual NCs are not perfectly spherical and exhibit a 10% size distribution. We have checked that, while the precise values fitted for c and R 0 are affected, the trends visible in Fig. 3e,f are robust to neglecting these geometrical details in the averaging procedure. For each solvent we determine the radiative decay rate γ rad from a maximum likelihood fit [34] of a single exponential to the data for LaPO 4 :Ce 3+ (1%) NCs. Subsequently, we fix γ rad in a global weighted least squares fit of equation 3 (with account for the different donor positions in an NC) to the data for the LaPO 4 :Ce 3+ (1%)Tb 3+ ( x %) NCs. How to cite this article: Rabouw, F. T. et al. Photonic effects on the Förster resonance energy transfer efficiency. Nat. Commun. 5:3610 doi: 10.1038/ncomms4610 (2014).